Interdependence of specialization and biodiversity in Phanerozoic marine invertebrates Studies of the dynamics of biodiversity often suggest that diversity has upper limits, but the complex interplay between ecological and evolutionary processes and the relative role of biotic and abiotic factors that set upper limits to diversity are poorly understood. Here we statistically assess the relationship between global biodiversity and the degree of habitat specialization of benthic marine invertebrates over the Phanerozoic eon. We show that variation in habitat specialization correlates positively with changes in global diversity, that is, times of high diversity coincide with more specialized faunas. We identify the diversity dynamics of specialists but not generalists, and origination rates but not extinction rates, as the main drivers of this ecological interdependence. Abiotic factors fail to show any significant relationship with specialization. Our findings suggest that the overall level of specialization and its fluctuations over evolutionary timescales are controlled by diversity-dependent processes—driven by interactions between organisms competing for finite resources. Recent methodological advances in the analysis of the fossil record and in the estimation of diversification rates from molecular phylogenies have enabled the refinement of global diversity curves [1] , [2] . These advances have also renewed and intensified interest in the nature of biodiversity dynamics—in terms of the importance of abiotic factors and biotic interactions as drivers of biodiversity and in tests of macroevolutionary hypotheses [3] , [4] , [5] , [6] , [7] . The hypothesis that global biodiversity has upper limits [8] is supported by evidence for diversity dependence of macroevolutionary rates [9] , [10] , [11] , slowdowns of speciation rates [4] , [7] and lack of a relationship between clade age and diversity [12] , [13] . Recent findings suggest that despite these saturation effects diversity can still increase, whereby ecological constraints slow down diversification [4] , [5] . A plausible explanation for an increase in diversity, even though ecospace is largely filled, would be provided by a diversity-dependent mechanism of niche subdivision, or increasing specialization. Indeed, interspecific competition constricts realized niches in extant species [14] , and low-diversity faunas in the fossil record are sometimes characterized by relatively high numbers of generalists (for example, refs 15 , 16 ). On the basis of these observations a relationship between diversity and specialization has been hypothesized [14] , [17] , [18] . Evidence for such a relationship is, however, only anecdotal and mainly restricted to times of low global biodiversity in the immediate aftermath of mass extinctions [16] , [19] . Little is known about the general validity of a relationship between diversity and specialization and about the underlying abiotic or biotic causes. Here we explore whether the temporal variation in habitat specialization of Phanerozoic marine invertebrates is related to diversity fluctuations and whether diversity affects origination probabilities of specialists and generalists. We use sampling-standardized occurrence data from the Paleobiology Database to estimate marine diversity and habitat specialization of genera in three major clades of benthic invertebrates—brachiopods, gastropods and bivalves. Habitat specialization of a genus is defined as a function of its realized ranges in three environmental categories, that is, water depth, substrate mineralogy and grain size of the substrate [18] . For example, a genus largely restricted to shallow-water and coarse-grained siliciclastic sediments is classified as a ‘true’ specialist, whereas a genus regularly occurring in shallow and deeper water, fine- and coarse-grained substrates, and siliciclastic and carbonate substrates is a ‘true’ generalist. Altogether, we distinguish between (1) all-category (‘true’) specialists, (2) one-category generalists, (3) two-category generalists and (4) three-category (‘true’) generalists. This approach provides a useful proxy for overall specialization, as a genus that inhabits different habitat types should also tolerate broader ranges of temperature, salinity, food availability and water energy. On the basis of origination rates, which were calculated for each of the four specialization groups, we estimated the degree of specialization of newly originated genera per time interval. Because ecological specialization and geographic range size are non-independent traits and both are closely linked to diversity [20] , [21] , [22] , [23] , [24] , [25] , this estimation involved the calculation of ‘partial’ regression coefficients (that is, ‘partial slopes’) in multiple linear regression models with geographic range size held constant. These partial slope values thus reflect the individual effect of habitat specialization on origination rates. Positive slopes indicate the preferential origination of specialists, the higher the values the more pronounced their habitat preference (see Methods for details). If there were indeed limits imposed on biodiversity and, once these limits are approached, a further increase in diversity was mediated by increasing specialization, then we would expect the overall specialization of the fauna to be positively correlated with standing diversity—locally, regionally and at a global scale. To test the validity of such a scenario we (1) determine variations in the proportions of specialists and the degree of specialization of new genera through time and test their correlation with diversity and (2) contrast the macroevolutionary rates of specialists and generalists for times of diversity increase and decrease. Our results provide evidence for a general feedback mechanism between biodiversity and the degree of ecological specialization. In times of high diversity, marine invertebrates are more specialized in their choice of preferred habitats. This subdivision of niche space is essentially controlled by above-average originations of specialists. Abiotic factors, specifically changes in sea level, nutrient availability, global climate and ocean oxygenation, do not show any significant relationship with specialization. These findings highlight the importance of diversity-dependent biotic interactions in shaping global marine diversity patterns on evolutionary timescales. Specialization and diversity Considering the three clades together, we find that origination probabilities are generally higher for specialists than for generalists, because slope values throughout the Phanerozoic eon are mostly positive ( Fig. 1a ). Moreover, the degree of specialization of newly originated genera and the proportion of specialists are positively correlated with genus-level diversity ( Fig. 1 ; Supplementary Tables 1–3 ). Correlation is stronger with the summed diversity of the three clades, but also evident with total marine diversity. This concordance is attributable to the overall similarity of the two diversity curves ( Supplementary Fig. 1 ), with brachiopods being a dominant element of Sepkoski’s ‘Palaeozoic evolutionary fauna’ and gastropods and bivalves dominating the ‘modern evolutionary fauna’ [26] . When the three clades are analysed separately, the proportions of specialists and the specialization of new genera are more strongly tied to diversity of the respective clade than to total marine diversity ( Supplementary Tables 2 and 3 ). 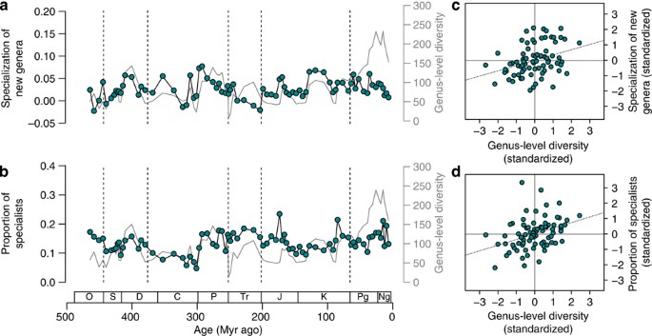Figure 1: Relationship between habitat specialization and diversity through the Phanerozoic. (a) Degree of specialization of newly originated genera in brachiopods, gastropods and bivalves. Values represent ‘partial slopes’ of the relationship between origination rates and specialization while controlling for potential effects of geographic range. Positive values indicate preferential origination of specialists over generalists, with higher values suggesting more pronounced preference. (b) Proportion of specialists within brachiopods, gastropods and bivalves. (c) Positive correlation between diversity and the degree of specialization of new genera (dotted line,n=79,ρ=0.37,P<0.001, Spearman’s rank correlation). (d) Positive correlation between diversity and the proportion of specialists (dotted line,n=79,ρ=0.41,P<0.001, Spearman’s rank correlation). Inaandb, the grey lines represent sampling-standardized summed diversity of the three clades; Phanerozoic mass extinctions are marked by dashed lines. Incandd, specialization indices and diversity estimates are detrended using residuals of smoothed time series, standardized to a mean of zero and unit s.d. Figure 1: Relationship between habitat specialization and diversity through the Phanerozoic. ( a ) Degree of specialization of newly originated genera in brachiopods, gastropods and bivalves. Values represent ‘partial slopes’ of the relationship between origination rates and specialization while controlling for potential effects of geographic range. Positive values indicate preferential origination of specialists over generalists, with higher values suggesting more pronounced preference. ( b ) Proportion of specialists within brachiopods, gastropods and bivalves. ( c ) Positive correlation between diversity and the degree of specialization of new genera (dotted line, n =79, ρ =0.37, P <0.001, Spearman’s rank correlation). ( d ) Positive correlation between diversity and the proportion of specialists (dotted line, n =79, ρ =0.41, P <0.001, Spearman’s rank correlation). In a and b , the grey lines represent sampling-standardized summed diversity of the three clades; Phanerozoic mass extinctions are marked by dashed lines. In c and d , specialization indices and diversity estimates are detrended using residuals of smoothed time series, standardized to a mean of zero and unit s.d. Full size image On average, the degree of specialization of newly originated genera in brachiopods, gastropods and bivalves is higher at times of high diversity than during periods of intermediate and low diversity ( Fig. 2 ). This suggests that, at high diversity, per-genus origination rates of specialists are above average and/or those of generalists are below average. However, additional factors may have contributed to the proportional increase of specialists, that is, lowered per-genus extinction rates of specialists and/or elevated per-genus extinction rates of generalists. Comparing times of diversity increase and decrease shows that intervals of increasing diversity are characterized by the preferential origination of specialists, while rates of generalists only play a secondary role ( Fig. 3a,b ). Diversity loss in all three clades is strongly linked to decreases in the origination rates of specialists and not to their (non-significant) elevated extinction rates. Again, rates of generalists exhibit only subtle changes ( Fig. 3c,d ). Thus, variation in the evolutionary dynamics of specialists, not generalists, determines diversity and the level of habitat specialization of the global marine biota. 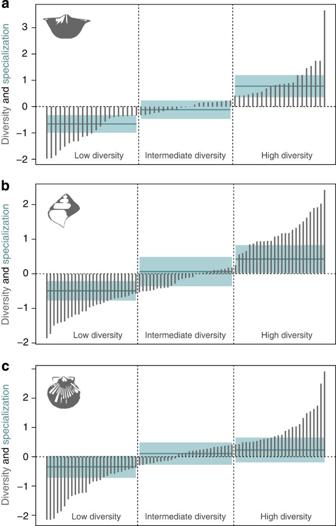Figure 2: Degree of habitat specialization of newly originated genera is correlated with diversity in marine Phanerozoic invertebrates. Within clades, average specialization of new genera is significantly higher during times of high diversity than during times of low diversity in brachiopods (a,n=42,P<0.001, Wilcoxon rank sum test) and gastropods (b,n=52,P<0.001) and marginally significant in bivalves (c,n=52,P=0.055). Vertical bars represent genus-level diversity across the Phanerozoic eon, ranked from lowest to highest. For statistical comparisons, we partitioned the values into three equally sized groups reflecting low, intermediate and high diversity, respectively. Blue horizontal lines indicate average degree of specialization of new genera for the different diversity levels, shaded areas represent 95% confidence intervals. Values of mean specialization and diversity are detrended using residuals of smoothed time series, standardized to a mean of zero and unit s.d. Figure 2: Degree of habitat specialization of newly originated genera is correlated with diversity in marine Phanerozoic invertebrates. Within clades, average specialization of new genera is significantly higher during times of high diversity than during times of low diversity in brachiopods ( a , n =42, P <0.001, Wilcoxon rank sum test) and gastropods ( b , n =52, P <0.001) and marginally significant in bivalves ( c , n =52, P =0.055). Vertical bars represent genus-level diversity across the Phanerozoic eon, ranked from lowest to highest. For statistical comparisons, we partitioned the values into three equally sized groups reflecting low, intermediate and high diversity, respectively. Blue horizontal lines indicate average degree of specialization of new genera for the different diversity levels, shaded areas represent 95% confidence intervals. Values of mean specialization and diversity are detrended using residuals of smoothed time series, standardized to a mean of zero and unit s.d. 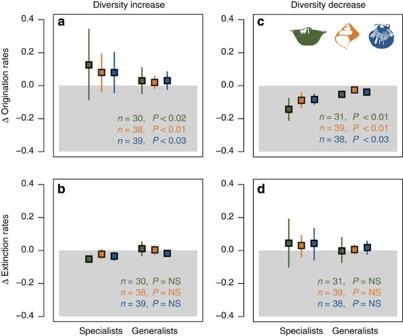Figure 3: Macroevolutionary rates of specialists and generalists in times of increasing and decreasing diversity. Elevated origination but not lowered extinction rates of specialists are linked to diversity increase in brachiopods (green), gastropods (orange) and bivalves (blue) (a,b). Decreases in diversity are associated with lowered origination rates of specialists, whereas elevated extinction rates are only of secondary importance (c,d). Under both diversity scenarios, changes in origination rates, but not in extinction rates, of specialists are significantly larger than in generalists (Wilcoxon paired-rank test). Error bars represent 95% confidence intervals.n, number of time intervals; NS, not significant. Full size image Figure 3: Macroevolutionary rates of specialists and generalists in times of increasing and decreasing diversity. Elevated origination but not lowered extinction rates of specialists are linked to diversity increase in brachiopods (green), gastropods (orange) and bivalves (blue) ( a , b ). Decreases in diversity are associated with lowered origination rates of specialists, whereas elevated extinction rates are only of secondary importance ( c , d ). Under both diversity scenarios, changes in origination rates, but not in extinction rates, of specialists are significantly larger than in generalists (Wilcoxon paired-rank test). Error bars represent 95% confidence intervals. n , number of time intervals; NS, not significant. Full size image Specialization and abiotic factors The observed diversity–specialization relationship does not per se allow conclusions about the underlying causes. Diversity and specialization could be controlling each other or they could have a common abiotic cause. Moreover, abiotic and biotic explanations for the observed general pattern may not be mutually exclusive. Various abiotic factors have been hypothesized as potential controls of diversity dynamics [27] and might also affect levels of specialization. In particular, it has been proposed that increased nutrient availability is associated with higher genus-level origination rates in the marine realm [28] , and a positive relationship between standing diversity and global temperature has been demonstrated throughout the Phanerozoic [29] . Furthermore, changes in sea level determine the amount of shallow water versus deeper water continental shelf area available for colonization [30] . Because the distribution of generalists and specialists in marine habitats is strongly depth related [31] , [32] , changes in sea level are a potential abiotic driver of changes in the degree of specialization. 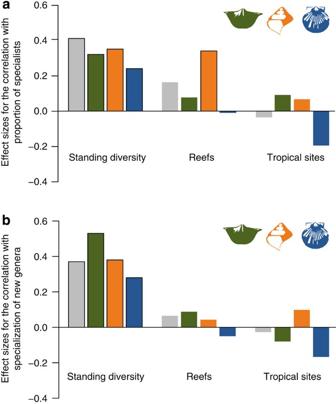Figure 4: Correlation between specialization and standing diversity, number of reefs and number of tropical sites through time. (a) In contrast to standing diversity, temporal variation in the proportion of reefs or tropical sites, as represented in the total marine data set, is not linked with the proportion of ‘true’ specialists in brachiopods (green), bivalves (blue) and in the summed data set (grey). Only in gastropods (orange) the proportion of ‘true’ specialists is closely associated with the number of fossil collections from reefs. (b) In contrast to standing diversity, the specialization of new genera is not significantly correlated with the proportions of collections coming from reefs or the tropics in any of the three clades. Bars inaandbrepresent effect sizes of Spearman’s rank correlations (that is, Spearman’s rho) between specialization and standing diversity of the respective clade and the proportions of collections from the respective environmental categories (n=79, except for brachiopods, wheren=63). Bars framed in black mark significant associations. All other associations are non-significant (P>0.05). We use a data set ( Supplementary Table 4 ) with estimates of eustatic sea level and isotopic proxies for environmental variables, specifically δ 18 O (proxy for temperature, although during icehouse conditions it also reflects ice volume), δ 13 C (proxy for changes in the carbon cycle), 87 Sr/ 86 Sr (proxy for inorganic nutrient input) and δ 34 S (proxy for organic nutrient input or shelf redox conditions) to test for a possible correlation between these environmental parameters and the proportion of ‘true’ specialists. We find no significant correlations between any of the potential abiotic controls and the proportion of ‘true’ specialists, either in the summed analyses or in separate analyses on brachiopods, gastropods and bivalves ( Table 1 ). Table 1 Association between proportion of ‘true’ specialists and eustatic sea level as well as other abiotic factors, assessed via the isotopic signatures of δ 18 O, δ 13 C, 87 Sr/ 86 Sr and δ 34 S, through time. Full size table Specialization and the distribution of habitats The positive correlation between specialization and standing diversity could simply arise from temporal variations in the number of fossil collections from environments known to harbour highly diverse and specialized faunas, such as reefs or the tropics [33] , [34] . Temporal variation in the extent of reefs or in the area of tropical seas might thus create an apparent change in diversity and specialization. This scenario would apply regardless of whether the fluctuations are attributable to the varying representation of reefs or tropical sites in the fossil record (that is, a sampling bias) or to true temporal variation in their distribution (that is, the pattern would be environmentally driven). We therefore tested for a possible correlation between specialization indices and the proportion of fossil collections from reefs and from tropical sites, respectively. We find that fluctuations through time in the proportion of reefal or tropical sites do not generally drive the observed fluctuations in specialization ( Fig. 4 ). Merely the proportion of ‘true’ specialists in gastropods is closely linked to the number of collections from reefs ( Fig. 4a ), whereas the specialization of genera that newly originate is not significantly correlated with the number of reefal or tropical collections in any of the three clades ( Fig. 4b ). The direction of a relationship between the number of collections from tropical sites and the specialization of newly originated bivalve genera, also evident in the proportion of ‘true’ specialists, would even be counter-intuitive to the discussed scenario. Overall, convincing evidence in support of the environmentally driven scenarios is lacking. Figure 4: Correlation between specialization and standing diversity, number of reefs and number of tropical sites through time. ( a ) In contrast to standing diversity, temporal variation in the proportion of reefs or tropical sites, as represented in the total marine data set, is not linked with the proportion of ‘true’ specialists in brachiopods (green), bivalves (blue) and in the summed data set (grey). Only in gastropods (orange) the proportion of ‘true’ specialists is closely associated with the number of fossil collections from reefs. ( b ) In contrast to standing diversity, the specialization of new genera is not significantly correlated with the proportions of collections coming from reefs or the tropics in any of the three clades. Bars in a and b represent effect sizes of Spearman’s rank correlations (that is, Spearman’s rho) between specialization and standing diversity of the respective clade and the proportions of collections from the respective environmental categories ( n =79, except for brachiopods, where n =63). Bars framed in black mark significant associations. All other associations are non-significant ( P >0.05). Full size image Excluding potential biases Fossil-based estimates of marine diversity can be distorted by heterogeneities in the rock record and changing preservation probabilities within different sedimentary environments through time [8] , [35] , [36] . We use subsampling procedures that explicitly account for sampling biases (see Methods), and that should minimize the effects of potential biases on diversity patterns. Yet, a biased rock record could still influence our perception of habitat specialization of the sampled taxa. For example, low preservation probabilities in particular environments would reduce a genus’ chance of being categorized as a ‘true’ generalist and enhance its chance of being categorized as a ‘true’ specialist. Therefore we tested for correlations between the proportion of ‘true’ specialists and preservation probabilities of taxa through time, both overall and within the different sedimentary environments used for the definition of habitat specialization herein. In the summed analyses on brachiopods, gastropods and bivalves, we find no significant correlations between the proportion of ‘true’ specialists and preservation probabilities of taxa through time, either with the overall preservation probability or with the probabilities within the different sedimentary environments ( Supplementary Table 5 ). Likewise, separate analyses on brachiopods and bivalves did not yield any significant results. Gastropods, in contrast, show a significant positive correlation between preservation probability and the proportion of ‘true’ specialists in shallow-water sediments. Although this link may affect the relationship between standing diversity and specialization in gastropods, it does not suffice to explain the overall patterns we found. Taxonomic practice and the use of outdated taxonomic identifications is another potential source of bias. Most genera in the fossil record are rare, whereas few very common ones contribute disproportionately to the total occurrence count. This hollow curve of abundance distributions might reflect a true biological signal but could also be influenced by taxonomic practice, in particular the lumping of taxa into ‘taxonomic wastebaskets’ [37] . Owing to their high abundance and commonly large geographic range, they are likely to be categorized as generalists, whereas the 'true' taxa that are lumped into a wastebasket taxon might have been more specialized. To assess whether potential candidates for wastebaskets affect the observed relationship between diversity and specialization, we excluded the 10 and the 20 most common taxa ( Supplementary Table 6 ) in each taxonomic group prior to the estimation of specialization indices and compared the resulting trajectories with those obtained including all genera. All curves are highly similar to each other, and the various specialization indices in summed and separate analyses are strongly positively correlated ( Supplementary Fig. 2 ). It is therefore highly unlikely that potential shortcomings in taxonomic practice affect our main results. In sum, we find that the relationship between standing diversity and specialization is not driven by systematic biases in the fossil and rock record, meaning that we can discuss our results in an evolutionary context. Our findings support and advance several general hypotheses in evolutionary biology. They corroborate earlier work suggesting that high ecological specialization is related to elevated rates of speciation [20] , [21] , [38] , [39] as well as the notion that losses in diversity can be driven by a lack of origination [6] , [40] . Furthermore, they confirm a general positive relationship between standing diversity and specialization and thus contribute to the ongoing debate on the role of biotic and abiotic factors as primary drivers of biodiversity dynamics. This debate has been dichotomized into two hypotheses, namely the Red Queen (biotic factors) and the Court Jester (abiotic factors). Irrespective of recent criticism of the Red Queen metaphor as a general description of evolutionary dynamics [41] , a consensus is forming that biotic and abiotic aspects are not mutually exclusive [3] , [11] , [42] . For example, the speciation of Cenozoic planktonic foraminifera was more strongly shaped by biotic variables than abiotic change, whereas the opposite was true for extinction [42] . Also, equilibrium or saturation models [1] , [8] , [10] , [43] , [44] propose the existence of equilibrium carrying capacities at which new taxa can only emerge at the expense of others. These models therefore imply a strong biotic control on global biodiversity, while the carrying capacity itself is determined by both the diversity-dependent strength of interactions and abiotic resource levels [5] , [28] , [45] . Such a biotic control on global biodiversity is supported by our results, whereas our analyses negate abiotic variables as drivers of the diversity–specialization relationship. We propose a feedback mechanism between standing diversity and specialization. Once ecospace is largely filled and saturation is approached with respect to the existing level of specialization, a further increase in diversity is mediated by niche subdivision, with finer subdivision being related to above-average origination of specialists. This mutually reinforcing coupling of diversity and partitioning of niche axes will continue—either until the differentiation of niche space is exhausted or until environmental turmoil results in extinctions and a drop in diversity. A biotic control on diversification patterns is further backed up by the evolutionary dynamics in the invertebrate groups that we studied. We find a stronger correlation between specialization and standing diversity within the respective clades than with total marine diversity ( Supplementary Tables 2 and 3 ). These clade-specific characteristics may well be explained by enhanced competition among closely related lineages for the same resources. Our results underscore the diversity-dependent origination rates of specialists as a principal controlling factor of global diversity. Apart from this evolutionary process, increasing competition could also force taxa towards their ecological optima, thereby contracting their realized habitat breadth without involving evolutionary adaptation. In a recently proposed model of diversity partitioning in competition-controlled systems [46] , this process defines the ‘habitat contraction phase’ and chronologically precedes the ‘niche differentiation phase’. Whether this purely ecological habitat contraction contributes to the observed diversity–specialization relationship remains to be tested with spatially and temporally more finely resolved data at the community level. Such studies could also address the issue to which degree taxa occur in sympatry, which is a prerequisite for any scenario involving competition. Meanwhile, we assume that the global patterns of the present analyses are a fair representation of the sum of patterns at the local and regional levels, that is, the scales at which competition occurs. This study on benthic marine invertebrates provides evidence for a general role of biotic factors in shaping global diversity patterns over the Phanerozoic. Unifying macroevolutionary principles should be applicable to both the marine and the terrestrial realm, but it has proven difficult to expand equilibrium models to terrestrial clades [3] . Nevertheless, the specialization of the terrestrial biota at large temporal and spatial scales may follow a similar diversity-dependent dynamic. Taxonomic occurrence data and taxonomic scope Diversity curves, macroevolutionary rates and proxies for habitat specialization were obtained through sampling standardization of Ordovician to Neogene genus-level taxonomic occurrence data, downloaded on 10 May 2013 from the Paleobiology Database ( http://paleobiodb.org ). We restricted the download to non-tetrapod metazoan occurrences, excluded collections from terrestrial environments and excluded genera with qualifiers ‘aff.’, ‘cf.’, ‘ex gr.’, ‘sensu lato’, ‘?’, ‘informal’ or listed in quotation marks. Prior to our analyses, we removed some predominantly non-marine groups that are listed in marine collections, such as basommatophoran gastropods, unionid bivalves and insects. We treated subgenera as genera and multiple species of the same genus in a single collection as a single occurrence. The marine fossil record provides a variety of well-preserved and abundant groups, but not all are equally well qualified to study habitat specialization on large temporal and spatial scales. To obtain indices for specialization, we focus on three major clades of marine benthic macroinvertebrates—brachiopods, gastropods and bivalves. These three clades have a rich fossil record, possess a primarily benthic lifestyle and are widely distributed among the surveyed settings. Our analyses thus focus on benthic ecosystems, with most of the data representing level-bottom communities but also including data from reefs. Because partitioning higher taxa with different intrinsic rates of evolution into different habitat types may bias results [9] , [47] , we performed analyses for each taxonomic group separately, but also conducted analyses over all genera of the three clades to maximize sample size and time range. In addition, we calculated total global marine diversity by using seven major groups of animal phyla and classes that are represented in the database by an adequate number of occurrences (that is, anthozoans, trilobites, brachiopods, echinoderms, cephalopods, gastropods and bivalves), supplemented by a ‘miscellaneous’ category in which the remaining taxa were treated together. Occurrences were binned into 83 time intervals equivalent to geological stages, except for the late Early Ordovician to early Middle Ordovician and the Rhuddanian to Aeronian, where in each case two neighbouring stages were combined. The final data set included 368,017 taxonomic occurrences of 20,825 genera from 67,816 collections. The brachiopod, gastropod and bivalve subsets comprised 82,584 occurrences (2,854 genera), 52,997 occurrences (3,482 genera) and 94,209 occurrences (2,459 genera), respectively. Sampling standardization and diversity estimates Sampling standardization was performed using a variant of the ‘shareholder quorum’ method [2] , [11] , a method that produces a fairer estimate of taxonomic richness than classical rarefaction because variations in abundance distributions are explicitly taken into account. The subsampling procedure used herein involves drawing fossil occurrences until the summed total of frequencies (that is, coverage) of the resampled taxa meet a target (the ‘quorum’). Taxon frequencies are corrected with a variant of Good’s u , which employs counts of single-publication taxa instead of singletons [2] , [11] . Literature-based compilations of occurrence data introduce several biases that have to be dealt with using modified protocols. For example, it is advisable to perform dispersed sampling or taxonomically split sampling [11] . Here we follow Alroy [2] in computing separate standardized diversity curves for the three focus clades and summed them up to a composite diversity curve of brachiopods, gastropods and bivalves. Similarly, to assess total marine diversity, we summed up the individual diversity of the major marine animal groups as outlined above ( Supplementary Table 1 ). The separate diversity curves were computed with quorum levels set to 0.50. The number of subsampling trials per analysis was set to 100. Sampled-in-bin counts of genera were adjusted with the three-timer correction to eliminate residual sampling biases [1] , [10] . Following Alroy [2] , the correction was applied only if the subsampled data for a given bin included an average of at least five three-timers. Otherwise, the uncorrected subsampled data were used. Counts for intervals with single-publication taxa only were set to zero. Calculation of macroevolutionary rates We computed per-genus extinction and origination rates applying the method established by Foote [48] , [49] . Origination rates ( O ) and extinction rates ( E ) are calculated as: O =−ln [ N bt /( N Ft + N bt )] and E =−ln [ N bt /( N bL + N bt )], where N bt is the number of taxa crossing both the bottom and top boundaries of an interval, N bL is the number of taxa crossing the bottom boundary but going extinct in the interval and N Ft is the number of taxa originating in the interval and crossing its top boundary. In accordance with Foote [50] and Alroy [10] we did not standardize rates for interval duration. As the calculation of rates is based on boundary crossers, single-interval taxa are automatically excluded. Rates for brachiopods are calculated only until the Danian, owing to insufficient numbers within particular habitat categories in the rest of the Cenozoic. The separate analyses on brachiopods were thus only performed over 67 time intervals, all other analyses over the full range of 83 time intervals. Prior to subsequent analyses, we excluded the first two (Early to Middle Ordovician) and last two (Pliocene or Maastrichtian to Danian, respectively) intervals of the time series to reduce edge effects. Proxies for habitat specialization and geographic range Wide niche breadth or a generalized ecology have been considered a key predictor of longevity and of speciation rates [20] , [21] , [22] , [38] , [51] , and the same has consistently been shown for geographic range [23] , [24] , [25] , [52] , [53] , [54] , [55] , [56] . Because these traits are not independent, their effects should be decoupled to infer the relationship between specialization and biodiversity dynamics. Our estimation of the specialization of newly originated genera (see below) therefore accounts for potential effects of geographic range. Habitat specialization and geographic range of each genus were determined according to its environmental and geographic distribution. Because these distributions depend on preservation potential and sampling intensity, their estimation is based on the sampling-standardized data sets. We defined habitat specialization of a genus as a function of its potential to inhabit different cells in habitat space (that is, its inverse ‘environmental tolerance’) [18] . To this end, habitat specialization was characterized as the probability of sampling a genus in one out of two states in three environmental categories: water depth (shallow and deeper water), substrate type (carbonates and siliciclastics) and grain size of the substrate (fine grained and coarse grained) (see refs 18 , 57 for a detailed assignment of depositional environments and the various types of sedimentary rocks to these broad environmental categories). Using the distribution of fossil occurrences in the different settings, we infer the range of abiotic environments, and thus the ecological adaptations, of each genus. Substrate type and water depth, for example, are related to temperature, salinity, nutrient influx and water energy. We classified a genus occurring with a probability higher than 0.8 in only one setting as a specialist in the respective category. Otherwise it was classified as a generalist. This rather generous threshold was chosen to overcome potential biases owing to, for example, allochthony or inaccuracies in the primary data. Finally, we converted the properties of a genus in the individual environmental categories into a combined measure of habitat specialization by distinguishing between (1) all-category specialists, (2) one-category generalists, (3) two-category generalists and (4) three-category generalists (see Supplementary Fig. 3 for proportional genus-level diversity of the four specialization groups through time). Using an occurrence probability of 0.9 rather than 0.8 as the threshold in classifying genera does not affect our conclusions. The four diversity curves calculated with a threshold value of 0.8 ( Supplementary Fig. 3a–d ) are significantly correlated with those obtained with a threshold value of 0.9 ( ρ =0.976, 0.950, 0.724 and 0.922, respectively, n =79 and P <0.001 for all comparisons, Spearman’s rank correlations). Assigning each genus to only a single group makes the implicit assumption that the underlying trait is more or less conserved, which is supported by a number of studies documenting niche conservatism or conserved habitat breadth [18] , [58] , [59] and relatively stable substrate preferences in marine invertebrates [60] , [61] . Geographic range size was defined as the maximum great circle distance of a genus within a time interval. The underlying palaeocoordinates of its occurrences are based on plate tectonic rotation data supplied by C. Scotese, which are implemented into the Paleobiology Database download scripts; see refs 18 , 55 for more details. For multiple regression analyses, we split the continuous geographic variable into five geographic range categories (0–1,000 km, 1,001–5,000 km, 5,001–10,000 km, 10,001–15,000 km and 15,001–20,000 km). The categories represent roughly 5,000-km distance bins with only the first one being distinctly smaller to distinguish truly narrowly distributed genera. The degree of specialization of newly originated genera (that is, the overall degree of specialization of genera originating in the focal time bin) was estimated as described in Nürnberg and Aberhan [18] . This involved calculation of ‘partial’ regression coefficients (that is, ‘partial slopes’) in multiple linear regression models to assess the individual effect of habitat specialization on origination rates with geographic range size held constant. Accordingly, we calculated the degree of specialization of new genera applying a regression model θ = β 0 + β 1 x 1 + β 2 x 2 , where θ is a vector of origination rates, x 1 and x 2 are the corresponding vectors of habitat specialization and geographic range, β 0 represents the intercept and the coefficients (slope values) β 1 and β 2 indicate the direction and the strength of habitat specialization and geographic range, respectively, on origination rate. The partial slopes were determined for each stratigraphic interval separately by analysing origination rates within a matrix of 4 × 5 possible combinations of habitat specialization and range size categories, as defined above. The partial slope value β 1 is then used as a measure of the degree of habitat specialization of new genera through time in brachiopods, gastropods and bivalves. Positive partial slope values indicate the preferential origination of specialists, the higher the values the more pronounced their habitat preference (see Fig. 1 and Supplementary Table 1 ). Proxies for abiotic and environmental variables All proxy data for abiotic variables were taken from Cárdenas and Harries [28] . Because the values are given for time intervals of ~5 Myr, we recalculated values for the midpoints of geological stages [62] using linear interpolations ( Supplementary Table 4 ). Reefs were defined according to the collection’s description on depositional environments in the Paleobiology Database. The following categories were included: ‘basin reef’, ‘slope/ramp reef’, ‘perireef or subreef’, ‘platform/shelf-margin reef’, ‘intrashelf/intraplatform reef’, ‘reef’ and ‘buildup or bioherm’. Collections with palaeolatitudes up to 30° north or south were assigned to the tropics. Preservation probability To estimate preservation probability we used gap analysis [63] as applied by Foote [48] . Accordingly, the preservation probability ( R i ) of taxa within a time interval is calculated as: R i = X bt,samp / X bt , where X bt is the observed number of taxa known both before and after an interval and X bt,samp is the number of these taxa actually sampled during an interval. The estimation of preservation probabilities is based on the complete downloaded raw data set. Thus R i reflects the overall likelihood that a marine taxon is preserved, collected and eventually entered into the database. Analytical methods To assess the relationship between habitat specialization and biodiversity dynamics, we have analysed time series of genus-level diversity and macroevolutionary rates of the various taxonomically and ecologically defined groups. We (1) analysed the trajectories of the proportions of ‘true’ specialists (that is, all-category specialists) and ‘true’ generalists (that is, three-category generalists) through time; (2) determined variations in the degree of specialization of newly originated genera through time while controlling for potential effects of geographic range; (3) tested for associations between these specialization indices and standing diversity, as well as abiotic variables; and (4) contrasted the macroevolutionary rates of ‘true’ specialists and ‘true’ generalists for times of diversity increase and decrease. All analyses were conducted in the R programming environment [64] . Because our data are largely non-normally distributed, associations between variables were tested by the nonparametric Spearman’s rank correlation, and tests for differences were based on the Wilcoxon rank sum and Wilcoxon paired-rank tests. Correlation of the raw data was carried out to identify long-term trends. Overall, there are temporal trends in most studied variables (for example, diversity estimates, specialization indices, overall preservation probability, the number of fossil collections coming from tropical sites and isotopic proxies for δ 18 O and 87 Sr/ 86 Sr). To remove problems with time series autocorrelation, all analyses, except those on changes in macroevolutionary rates (see below), are based on detrended data. Variables were detrended using smoothing splines applying the function ‘smooth.spline’ in R with the default settings except for the degrees of freedom of the spline, which was set to 15. Residuals from the spline were then standardized to a mean of zero and unit s.d. ( z -scores) and used to test for associations between variables. This procedure removes long-term trends while retaining medium-term (multiple time bins) variability. Standardizing the detrended data facilitates interpretation of the plots because all variables use the same scale. We also detrended time series by taking generalized differences [65] ( Table 1 ; Supplementary Tables 3 and 5 ). While generalized differences are used in geological applications to test for short-term correlation in bin-to-bin shifts, residuals from the smoothing splines allow to evaluate differences in the studied variables relative to their values in (multiple) neighbouring time intervals. To contrast origination and extinction rates of ‘true’ specialists and ‘true’ generalists for times of diversity increase and decrease, we computed first differences (that is, changes between adjacent time intervals) to identify times of increasing and decreasing diversity and to determine the corresponding change in macroevolutionary rates. We note that, given their computation following Foote [48] , [49] , originations within a time bin contribute to the standing diversity of that same bin, while extinctions lower the standing diversity of the immediately following time interval. Thus, changes in extinction rates, in contrast to those in origination rates, are tied to subsequent changes in diversity. Therefore, calculated changes in origination rates were paired with simultaneous changes in diversity, whereas changes in extinction rates were paired with subsequent changes in diversity (see above for further details on diversity estimates and computation of per-genus origination and extinction rates). Accession codes : Fossil Occurrence Data are available from the Paleobiology Database ( http://paleobiodb.org ). How to cite this article: Nürnberg S. and Aberhan M. Interdependence of specialization and biodiversity in Phanerozoic marine invertebrates. Nat. Commun . 6:6602 doi: 10.1038/ncomms7602 (2015).